A protective layer approach to solvatochromic sensors As they have been designed to undergo colorimetric changes that are dependent on the polarity of solvents, the majority of conventional solvatochromic molecule based sensor systems inevitably display broad overlaps in their absorption and emission bands. As a result, colorimetric differentiation of solvents of similar polarity has been extremely difficult. Here we present a tailor-made colorimetric and fluorescence turn-on type solvatochromic sensor that enables facile identification of a specific solvent. The sensor system displays a colorimetric transition only when a thin protective layer, which protects the solvatochromic materials, is destroyed or disrupted by a specific solvent. The versatility of the strategy is demonstrated by designing a sensor that differentiates chloroform and dichloromethane colorimetrically and one that performs sequence selective colorimetric sensing. In addition, the approach is employed to construct a solvatochromic molecular AND logic gate. The new strategy could open new avenues for the development of novel solvatochromic sensors. A challenging task in chemistry has been the development of a solvatochromic sensor that is responsive to a specific solvent. Various organic [1] , [2] , [3] , [4] , [5] , [6] , [7] , [8] , [9] , [10] , organometallic [11] , [12] , metal organic framework [13] , [14] and hybrid [15] , [16] materials have been investigated to determine their solvatochromic properties in diverse solvents. Conventional colorimetric sensors, however, inevitably display changes in absorption and emission peaks that are in indiscriminant in their response to organic solvents. This phenomenon is a consequence of the fact that the probe molecules are designed to undergo spectral shifts that depend solely on the polarity of surrounding medium. Because of this limitation, visual differentiation of solvents that have similar polarities has been very difficult. In this study, we devise a new approach to designing a system for colorimetric differentiation of common organic solvents. The new tailor-made colorimetric and fluorescence turn-on type solvent sensor system enables facile naked eye identification of one among several solvents. The key strategy employed for the sensor system is schematically described in Fig. 1a . A solvatochromic material is first coated on a solid substrate and then covered with a thin protective layer. As a result, the solvatochromic sensor molecules are protected from direct exposure to organic solvents unless the solvent disrupts the protective layer by either dissolution or swelling. In the latter event, the solvatochromic molecules are exposed to the solvent and undergo an observable colorimetric transition. As the colorimetric transition of the sensor system is dependent on the properties of the protective layer and the solvent, it does not require that the solvatochromic substance respond in a specific manner to a certain solvent. By using the new approach, we devise a system that is able to distinguish between dichloromethane and chloroform, two solvents that are very difficult to differentiate colorimetrically. In addition, the new solvatochromic strategy is used to fabricate a sequence selective solvatochromic sensor as well as a colorimetric AND logic gate [17] , [18] , [19] , [20] , [21] , [22] , [23] , [24] . The significant features of the solvatochromic sensor system developed in this study are as follows. First, the colorimetric signal generated upon exposure of the system to a specific target solvent is easily recognized by using the naked eye. Second, a single solvatochromic dye can be employed in systems that differentiate several different solvents. Third, commercially available and inexpensive polymers can be used as the protective layers. Fourth, the sensor film can be readily fabricated by utilizing simple spin-coating or drop-casting techniques. Fifth, colorimetric changes of the sensor film occur in most cases within 1 min of exposure to the solvent. Finally, the strategy can be employed in the preparation of a variety of tailor-made sensors that are comprised of properly selected dyes and protective layers. 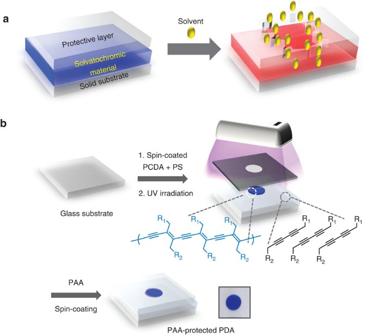Figure 1: Fabrication of the solvatochromic sensor system. (a) Schematic representation of the colorimetric sensor system. (b) Fabrication of polyacrylic acid (PAA)-protected polydiacetylene (PDA) film on a glass substrate. Figure 1: Fabrication of the solvatochromic sensor system. ( a ) Schematic representation of the colorimetric sensor system. ( b ) Fabrication of polyacrylic acid (PAA)-protected polydiacetylene (PDA) film on a glass substrate. Full size image Colorimetric and fluorescence turn-on sensor In order to determine the feasibility of the turn-on solvatochromic sensor strategy described above, studies were carried out using the conjugated polydiacetylene (PDA) polymer [25] , [26] , [27] , [28] , [29] , [30] , [31] , [32] , [33] , [34] , [35] , [36] , [37] , [38] , [39] derived from 10,12-pentacosadiynoic acid (PCDA, CH 3 (CH 2 ) 11 C≡C−C≡C(CH 2 ) 8 COOH), which is a well-known solvatochromic material ( Supplementary Fig. S1 ). A thin film ( ca. 1.0 μm) was prepared on a glass substrate by first spin-coating a viscous solution PCDA (40 mg ml −1 ) and polystyrene (PS, Mw: 280,000 g mol −1 ) ( Fig. 1b ) followed by irradiation with UV light (254 nm, 1 mW cm −2 , 3 min) to induce polymerization. As a photomask was used in the irradiation step, blue-phase PDAs are generated only in UV-exposed areas. Finally, the generated PDA film was coated to a thickness of ca. 1.5 μm using a methanol solution of poly(acrylic acid) (PAA, Mw: 450,000 g mol −1 ). As neither PS nor PDA is soluble in water, the PS film containing PDA is stable during the PAA coating process. Implementation of this simple procedure led to fabrication of a PAA-protected blue-phase PDA film on a glass substrate. Very interesting observations were made when pipette drops ( ca. 100 μl) of common organic solvents were applied to the tops of unprotected and PAA-protected PDA films ( Fig. 2a ). As expected, unprotected PS films containing PDAs undergo an observable colour changes when exposed to most of the tested solvents, except for methyl alcohol (MeOH), isopropyl alcohol (IPA), hexane and acetonitrile (ACN) ( Fig. 2a , top). In contrast, when the PAA-protected PDA films were exposed to the solvents, only the one treated with tetrahydrofuran (THF) undergoes a blue-to-red colorimetric transition ( Fig. 2a , middle) (see also Supplementary Movie 1 ). As the red coloured form of the PDA is fluorescent while the blue counterpart is virtually nonfluorescent [40] , [41] , only the THF-exposed film emits red fluorescence ( Fig. 2a , bottom). Visible absorption spectra of the PAA-coated PDA films were also recorded after exposure to the solvents. A significant spectral shift associated with the blue-to-red transition was observed to take place only with the film that was treated with THF ( Fig. 2b ). The chemical nature of the colour change process was also probed by using Raman spectroscopy ( Supplementary Fig. S2 ). The conjugated alkyne–alkene groups in the Raman spectrum of the blue-phase PDA appear at 2081 (C≡C) and 1,451 cm −1 (C=C) [42] . Inspection of the Raman spectrum of the red-phase PDA, obtained by exposure of the film to THF, shows that the alkyne–alkene bands at 2,081 and 1,451 cm −1 are shifted to higher frequencies (2,121 and 1,515 cm −1 , respectively). This finding demonstrates that most of the blue-phase PDAs are transformed to red-phase counterparts upon THF treatment. 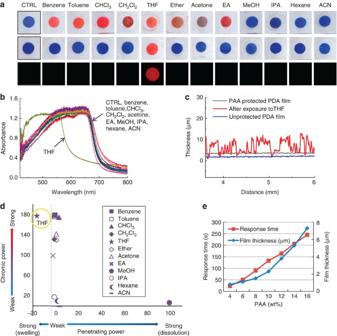Figure 2: THF-specific solvatochromism. (a) Photographs of solvent-exposed unprotected (top) and PAA-protected (middle) PCDA-derived PDA films. Fluorescence microscope images of the solvent-treated PAA-protected PDA film are also displayed (bottom). Photographs were taken 1 min after adding a drop (ca.100 μl) of each solvent to the top of the film. (b) Absorption spectra of PAA-protected PDA film upon exposure to various solvents. (c) Film thickness as a function of distance before (blue line) and after (black line) PAA protection. The fluctuating red line is obtained after exposure of the PAA-protected PDA film to THF. (d) Plots of PDA chromic power versus PAA penetrating power for various solvents tested. (e) Plots of colorimetric response time and film thickness as a function of concentration of protective PAA. Figure 2: THF-specific solvatochromism. ( a ) Photographs of solvent-exposed unprotected (top) and PAA-protected (middle) PCDA-derived PDA films. Fluorescence microscope images of the solvent-treated PAA-protected PDA film are also displayed (bottom). Photographs were taken 1 min after adding a drop ( ca. 100 μl) of each solvent to the top of the film. ( b ) Absorption spectra of PAA-protected PDA film upon exposure to various solvents. ( c ) Film thickness as a function of distance before (blue line) and after (black line) PAA protection. The fluctuating red line is obtained after exposure of the PAA-protected PDA film to THF. ( d ) Plots of PDA chromic power versus PAA penetrating power for various solvents tested. ( e ) Plots of colorimetric response time and film thickness as a function of concentration of protective PAA. Full size image Two critical factors must be considered when deciphering the solvatochromic behaviour of the PAA-protected PDA film described above. The film disrupting power of the solvent caused by dissolution and/or swelling is one important parameter, because these processes must occur in order for solvent molecules to reach and interact with the PDAs. PAA layer disruption was demonstrated by determining the thickness profile of the film before and after exposure to solvents. The results show that a significant disruption of the sensor film occurs when it is placed in contact with THF ( Fig. 2c ) but that this phenomenon does not take place when other solvents, except MeOH, are used ( Supplementary Fig. S3 ). The layer disrupting power of a solvent can also be evaluated by measuring the weights of a PAA-coated film before and after incubation in a solvent ( Supplementary Fig. S4 ). The results of these measurements show that no significant change in weight takes place for films treated with all tested solvents except MeOH and THF. In the presence of MeOH, PAA layer is nearly completely removed while the weight of THF-treated PAA film increases by 16.4% after incubation in THF. The latter observation indicates that immobilization of THF molecules occurs in the film. The other critical factor responsible for promoting the colorimetric transition is the ability of the solvent to induce the blue-to-red associated phase transition of the PDA molecules ( Supplementary Fig. S5 ). The colorimetric change inducing ability of each solvent, displayed in Supplementary Fig. S5 , was determined by measuring the intensity of the red colour developed when the unprotected PDA film is exposed to each solvent. The results show that not all solvents, which penetrate the protective PAA layer, are capable of inducing the blue-to-red colour transition. For instance, MeOH readily dissolves the hydrophilic PAA layer but it is ineffective in promoting the phase change of the PDA supramolecules in the film state. It should be noted that incubation of the PDA powder alone in MeOH causes a blue-to-purple colour change ( Supplementary Fig. S1 ), a finding that indicates that the hydrophobic PS matrix used for the fabrication of PDA film serves as a protective layer repelling hydrophilic MeOH. Inspection of Fig. 2d , in which a plot correlating the two important parameters related to colorimetric response and penetrating ability is given, demonstrates that these parameters are well related to the solvent specific colorimetric changes depicted in Fig. 2a . Specifically, because THF has both strong colorimetric and film penetrating (by swelling) properties in contrast to other solvents, it can be selectively identified by using a properly designed colorimetric and fluorescence turn-on type THF selective solvatochromic sensor system. The protective layer strategy also enables manipulation of the colorimetric response time of the sensor film. For instance, the thickness of the protective layer can be readily controlled by varying either the concentration of the protective polymer solution or the number of spin-coating using a fixed concentration of the polymer solution ( Supplementary Figs S6 and S7 ). This expectation is confirmed by the results displayed in Fig. 2e , which show that the thickness of the protective layer increases as the concentration of PAA increases. Importantly, as time is required for the THF molecule to disrupt the PAA layer and reach the solvatochromic PDA layer, the response time for promotion of the blue-to-red colour transition increases as the thickness of the protective layer increases. In order to address important sensitivity related issues with regard to the solvatochromic sensor system, additional experiments were carried out. It is obvious that if the diameter of the sensor spot exposed to the organic solvent is smaller, a lower amount of the solvent would be required to promote the colorimetric transition. Interestingly, additional studies showed that only one microliter of THF is sufficient to cause the blue-to-red colour change of the polymer when a sensor spot of 2 mm diameter is employed ( Supplementary Fig. S8 ). In addition, the solvatochromic sensor system is also applicable to systems in which the solvent of interest is diluted with other solvent. To demonstrate this feature, solvatochromic tests were carried out on mixtures of THF and ACN. ACN was selected as a diluting solvent because it does not induce the colorimetric transition of the PDA and it is completely miscible with THF. We observed that the sensor system functions well for solutions up to a 50 vol% THF-ACN ( Supplementary Fig. S9 ). Regarding the detection limit in terms of time, we observed that the time required for the colorimetric response decreases as the thickness of the protective layer decreases ( Fig. 2e ). In addition, if the protective layer is too thin (below a micrometre), no colorimetric selectivity is achieved for the THF sensor due to the loss of the function of the protective layer. Thus, minimum contact time required for good solvatochromic discrimination is ca. 20 s. Differentiation between chloroform and dichloromethane We next investigated the design of a more challenging sensor system that is capable of distinguishing between the very closely related solvents, chloroform and dichloromethane. Supplementary Fig. S1 shows that both chloroform and dichloromethane bring about an indistinguishable blue-to-red colour change when they are individually applied to the PCDA-derived PDA powder. Thus, we anticipated that the protective layer approach could be used to carry out the challenging visual differentiation between these two solvents. Among various commercially available polymers, poly(vinylchloride) (PVC) has a strikingly different solubility in the two solvents, being highly soluble in dichloromethane and only poorly soluble in chloroform ( Fig. 3d , Supplementary Fig. S10 ). Consequently, these two solvents should be colorimetrically distinguishable when PVC is used as the protective layer. In order to test this proposal, a sensor system, created by using a modified double-layer protection approach, was prepared ( Fig. 3a ). First, a thin PS film containing the PDA was applied to a glass substrate (as described in Fig. 1b ). Second, spin-coating a MeOH solution containing polyvinylpyrrolidone (PVP, Mw: 360,000 g mol −1 , 12 wt%) afforded a thin PVP layer on the top of the PDA film. The coating of PVP, which is highly soluble in both chloroform and dichloromethane ( Supplementary Fig. S11 ), is required as a ‘dummy’ layer in this case because direct coating of PVC on the top of the PDA causes disruption the PDA supramolecules and a premature blue-to-red colorimetric change of the polymer film. Finally, the solvent distinguishable PVC layer was introduced on top of the PVP film by spin-coating a THF solution (12 wt%) containing this polymer (Mw: 620,000 g mol −1 ). 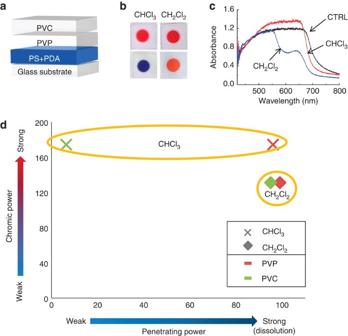Figure 3: Colorimetric differentiation between dichloromethane and chloroform. (a) Schematic of a double-layer protected sensor system. (b) Photographs of solvent-exposed single- (top, PVC), and double- (bottom, PVC-on-PVP) layer protected PCDA-derived PDA films. Photographs were taken 1 min after adding a drop (ca. 100 μl) of each solvent to the top of the film. (c) Absorption spectra of double-layer protected PDA films upon exposure to chloroform and dichloromethane. (d) Plots of PDA chromic power versus layer penetrating power for chloroform and dichloromethane. Figure 3: Colorimetric differentiation between dichloromethane and chloroform. ( a ) Schematic of a double-layer protected sensor system. ( b ) Photographs of solvent-exposed single- (top, PVC), and double- (bottom, PVC-on-PVP) layer protected PCDA-derived PDA films. Photographs were taken 1 min after adding a drop ( ca . 100 μl) of each solvent to the top of the film. ( c ) Absorption spectra of double-layer protected PDA films upon exposure to chloroform and dichloromethane. ( d ) Plots of PDA chromic power versus layer penetrating power for chloroform and dichloromethane. Full size image When individually applied, both chloroform and dichloromethane induce an immediate blue-to-red colour change of a polymer film comprised of the upper ‘dummy’ PVP and lower sensing PDA layer ( Fig. 3b , top). In contrast, individual application of the two solvents to the PVC-protected film results in completely different outcomes. The dichloromethane-treated film undergoes a colour transition to red while the chloroform-treated sample does not experience a colour change ( Fig. 3b , bottom) (see also Supplementary Movie 2 ). Absorption spectroscopic monitoring of these processes ( Fig. 3c ) has also been used to follow the changes occurring in the solvent and protective layer dependent processes. Consequently, because both chloroform and dichloromethane have a strong colorimetric transition power for PDA, their different abilities to solubilize PVC can be utilized as the basis for a dichloromethane-selective colorimetric sensor system. IPA selective solvatochromic sensor During the course of this study, we observed that an unprotected PDA film derived from 10,12-tricosadiynoic acid (TCDA, CH 3 (CH 2 ) 9 C≡C–C≡C(CH 2 ) 8 COOH) undergoes a blue-to-red colorimetric transition when treated with alcoholic solvents such as MeOH and IPA ( Supplementary Fig. S12 ). TCDA contains a two carbon shorter alkyl chain than PCDA, which makes the colour transition of the TCDA-derived polymer more sensitive to alcoholic solvents than the polymer derived from PCDA, which does not undergo a MeOH or IPA promoted colorimetric transition when a incorporated in a PS film ( Fig. 2a , top). These observations led to the design an IPA selective solvatochromic sensor. A double-layer protected sensor film, comprised of (PVP/PAA/PDA), was constructed for this purpose. As expected, the unprotected TCDA-derived PDA film undergoes a colour transition when treated with all of the tested solvents except hexane and ACN ( Fig. 4a ). In contrast, the single-layer (PAA) protected film is only highly colorimetrically responsive to IPA and THF and to a lesser extent MeOH and acetone, owing to the polar nature of the PAA matrix ( Fig. 4b ). Finally, only IPA is able to penetrate the double-layer protected sensor film and cause a blue-to-red colour change of the burried PDA supramolecules ( Fig. 4c ). 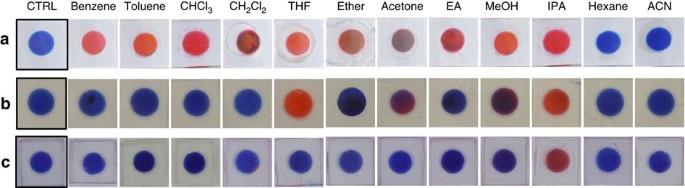Figure 4: IPA selective solvatochromic sensor. (a–c) Photographs of the solvent-exposed unprotected (a), single-layer protected (PAA/PDA) (b) and double-layer protected (PVP/PAA/PDA) (c) TCDA-derived PDA films. Photographs were taken 1 min after dropping each solvent on the top of the film. Figure 4: IPA selective solvatochromic sensor. ( a – c ) Photographs of the solvent-exposed unprotected ( a ), single-layer protected (PAA/PDA) ( b ) and double-layer protected (PVP/PAA/PDA) ( c ) TCDA-derived PDA films. Photographs were taken 1 min after dropping each solvent on the top of the film. Full size image Solvatochtomic logic circuits One unique advantage of the protective layer approach to solvent identification not found in conventional film or solution-based sensors is that it enables construction of a sequence selective sensor system. We observed that a poly(methyl methacrylate) (PMMA) and PVP-protected PCDA-derived PDA film ( Fig. 5a ) responds to two solvents in a sequence selective manner. Accordingly, a blue-to-red colour transition occurs when this film is exposed sequentially to IPA and toluene ( Fig. 5b ) but a colour change does not take place when the sensor film is treated in a reverse sequential manner (that is, toluene first) with these solvents. The solubility differences of the two protective polymers, PVP and PMMA, in IPA versus toluene is responsible for this sequence selective solvatochromic behaviour. Application of IPA to the sensor film results in removal of the PVP layer owing to the solubility of this polymer in alcoholic solvents ( Supplementary Fig. S11 ). The thickness profile data presented in Fig. 5d demonstrate this property. In the initial constructing stage, the thickness of the sensor film increases sequentially as PMMA (1st layer) (blue line) and PVP (2nd layer) (green line) layers are coated on the top of the PDA polymer film (black line). Exposure of the resulting film to IPA causes a decrease in the thickness of the PMMA layer (red line), but toluene is ineffective in disrupting/dissolving the PVP layer. However, owing to its solubilizing properties toluene easily penetrates the PMMA layer so that it can induce colorimetric transition of the polymeric PDA molecules ( Supplementary Fig. S13 ). 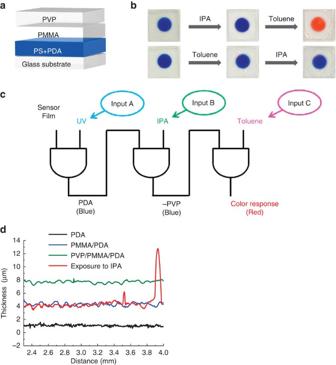Figure 5: Sequence selective logic gates. (a) Schematic of a double-layer protected PCDA-derived PDA film for a sequence-specific colorimetric sensor. (b) Photographs of the sensor films after exposure to IPA and toluene in different order. (c) A solvatochromic keypad lock logic circuit. (d) Film thickness as a function of distance before (black) and after protection with PMMA (blue) and PVP (green). The red line is obtained after exposure of the sensor film to IPA. Figure 5: Sequence selective logic gates. ( a ) Schematic of a double-layer protected PCDA-derived PDA film for a sequence-specific colorimetric sensor. ( b ) Photographs of the sensor films after exposure to IPA and toluene in different order. ( c ) A solvatochromic keypad lock logic circuit. ( d ) Film thickness as a function of distance before (black) and after protection with PMMA (blue) and PVP (green). The red line is obtained after exposure of the sensor film to IPA. Full size image These observations demonstrate that the protective layer approach can be used to fabricate a sensor system that displays the general mechanistic features of a keypad lock logic circuit [43] ( Fig. 5c ), in which UV irradiation, IPA and toluene inputs need to be applied in an ordered sequence in order to turn on the system ( Table 1 ). Another salient feature of the protective layer strategy is that it enables the design of solvatochromic molecular AND logic gates. For example, the sensor system displayed in Fig. 6a functions only when water and THF are present as input signals. No colour change occurs if the sensor film is exposed to water alone because the hydrophobic PVC layer is not soluble in this solvent ( Fig. 6b , top). In addition, even though it disrupts the top PVC layer, THF does not reach the sensor layer owing to poor penetrability through the poly(vinyl alcohol) (PVA) layer. As a result, no apparent colour change of the PCDA-derived PDA occurs ( Fig. 6b , middle). However, a blue-to-red colorimetric transition does take place when the sensor system is exposed to aqueous THF ( Fig. 6b , bottom) and, consequently, the sensor system serves as a two-input (H 2 O and THF) solvatochromic AND logic gate ( Fig. 6c , Table 2 ). It is significant to note that this sensor system functions well even when a 2 vol% H 2 O-THF solution is used ( Fig. 6d ), suggesting that it can be applied as sensitive colorimetric system to determine the anhydrous nature of solvents if more water sensitive protective layers are employed. Table 1 Truth table for the solvatochromic keypad lock system upon varying the order of the input signals. 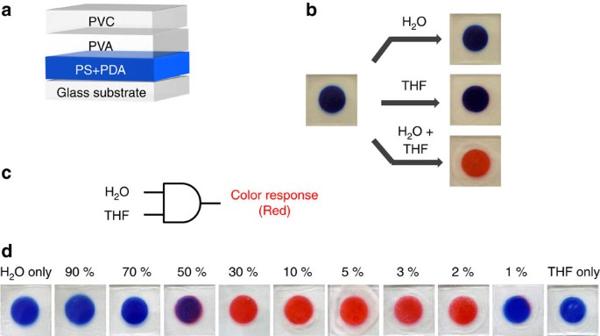Figure 6: Solvatochromic AND logic gates. (a) Schematic of a double-layer protected PCDA-derived PDA film for an AND logic gate. (b) Photographs of the sensor film after exposure to H2O, THF and 20% aqueous THF. (c) A two-input solvatochromic AND logic gate. (d) Colorimetric response of the sensor film after exposure to various volume compositions of water in THF. Full size table Figure 6: Solvatochromic AND logic gates. ( a ) Schematic of a double-layer protected PCDA-derived PDA film for an AND logic gate. ( b ) Photographs of the sensor film after exposure to H 2 O, THF and 20% aqueous THF. ( c ) A two-input solvatochromic AND logic gate. ( d ) Colorimetric response of the sensor film after exposure to various volume compositions of water in THF. Full size image Table 2 Truth table for the two-input (H 2 O and THF) AND gate. Full size table Fluorescence turn-on sensor system The flexible nature of the protective layer strategy enables it to be applied to the design of turn-on sensors that contain target and response guided sensor matrixes. For example, the formation of a fluorescamine-primary amine adduct can be utilized for the fabrication of a solvent responsive fluorescence turn-on sensor ( Fig. 7 ). Fluorescamine is virtually nonfluorescent but it reacts with primary amines to generate strongly fluorescent adducts [44] . By taking advantage of this property, we have designed a novel layered fluorescence sensor system ( Fig. 7a ). A thin PS film containing fluorescamine, prepared on a glass substrate, was sequentially coated with a PVP layer and then a PMMA layer containing the primary amine, octadecylamine. Octadecylamine was selected for this purpose because its low volatility avoids losses that could occur during sensor preparation. In this device, the primary amine and fluorescamine are separated by the intervening PVP layer. We expected that disruption of the PVP layer by solvents would remove the barrier between two reactants and, thus, allow free diffusion and reaction between fluorescamine and amine. In Fig. 7b are shown vials containing fluorescamine and octadecylamine in the selected organic solvents toluene, chloroform, THF, ethyl acetate and methanol. Each vial emits blue adduct derived fluorescence upon irradiation with 365 nm UV light. To demonstrate the importance of the protective layer, a polymer film containing a PS-fluorescamine and PMMA-octadecylamine layer and not possessing an intervening PVP layer was prepared by using spin-coating. As can be seen in Fig. 7c , this film emits blue fluorescence under UV light (see also Supplementary Fig. S14 ). In contrast, the corresponding polymer film containing the intervening PVP protective layer displays no fluorescence emission (see also Supplementary Fig. S14 ). Exposure to chloroform results in the generation of a circled fluorescence pattern owing to the coffee ring effect that is generally observed with a liquid drop ( Fig. 7e ) [45] . The results obtained in this study of the fluorescamine- and octadecylamine-based film demonstrate that unique solvatochromic turn-on fluorescence sensor systems can be devised by simply choosing appropriate stimuli responsive molecules and protective layers. 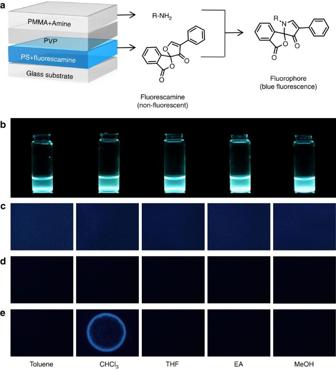Figure 7: A fluorescence turn-on solvatochromic sensor system. (a) Schematic representation of a fluorogenic sensor system based on fluorescamine-amine adduct formation. (b) Photographs of vials containing solutions of fluorescamine (2 mg ml−1) and amine (2 mg ml−1) under 365 nm UV light. (c) Photographs of unprotected films (without PVP layer) under 365 nm UV light. (d) Photographs of PVP-protected films under 365 nm UV light. (e) Photographs of PVP-protected films under 365 nm UV light after exposure to various solvents. Figure 7: A fluorescence turn-on solvatochromic sensor system. ( a ) Schematic representation of a fluorogenic sensor system based on fluorescamine-amine adduct formation. ( b ) Photographs of vials containing solutions of fluorescamine (2 mg ml −1 ) and amine (2 mg ml −1 ) under 365 nm UV light. ( c ) Photographs of unprotected films (without PVP layer) under 365 nm UV light. ( d ) Photographs of PVP-protected films under 365 nm UV light. ( e ) Photographs of PVP-protected films under 365 nm UV light after exposure to various solvents. Full size image PDAs undergo a distinct colour change (typically blue-to-red) when their arrayed p-orbitals are distorted under the influence of environmental perturbations and the observed change in colour is dependent on the degree of the distortion. As PDAs are formed from self-assembled diacetylene monomers, individual PDA chain interacts strongly with neighbouring PDAs, a feature that makes most PDAs insoluble in most solvents. When solvent molecules disrupt the densely packed PDA chains that cause an increase in the interchain distance, a colorimetric transition occurs as a result of the partial distortion of the p-orbital overlap. If individual PDA chains are separated by their individual interactions with a good solvent, the resulting severe distortion of the conjugated p-orbital array results in a blue-to-yellow colour transition. But the poor solubility of PDAs in most organic solvents leads to a lower degree of distortion and, consequently, a blue-to-red (or purple) colour change. PDA supramolecules derived from a single chain diacetylene that contains a terminal carboxylic acid (for example, PCDA) display a solvent nonspecific colour change when they are exposed to common organic solvents. The study described above has demonstrated the viability and generality of a new solvatochromic sensor strategy. By taking advantage of the protective layer approach, we were able to devise unprecedented colorimetric and fluorescence turn-on type solvatochromic film sensors that carry out the demanding task of visual differentiation of solvents. The source of the selectivity of this type of sensor resides in a colorimetric transition of solvatochromic molecules that only occur when a target solvent disrupts a properly selected protecting layer. The PAA-protected PDA system clearly demonstrates that a tailor-made THF-specific colorimetric sensor can be fabricated. In addition, by taking advantage of the protective layer approach, we were able to devise a sensor that carries out the demanding task of colorimtrically distinguishing between dichloromethane and chloroform. Facile fabrication of a sensor system that has solvent sequence selectivity as well as ready construction of a solvatochromic molecular AND logic gate are additional meritorious features of employing the protective layer-based sensor strategy. Finally, the flexibility of the protective layer approach was further demonstrated by constructing a system, which relies on a fluorescamine-amine adduct forming reaction, for solvent-selective fluorescence turn-on sensing. It is believed that the new strategy developed in this effort will find wide application in the design of tailor-made solvatochromic chemosensors. Materials and instruments 10,12-Pentacosadiynoic acid (PCDA) and TCDA were purchased from GFS Chemicals, Ohio, USA. PAA (Mw: 450,000 g mol −1 ), PVP (Mw: 360,000 g mol −1 ), PVC (Mw: 620,000 g mol −1 ), PMMA (Mw: 120,000 g mol −1 ), poly(ethylene oxide) (Mw: 200,000 g mol −1 ) and poly(vinyl alcohol) (PVA, Mw: 89,000–98,000 g mol −1 ), used as protective layers, were obtained from Aldrich Co. Fluorescamine and octadecylamine were purchased from Aldrich Co. Spectroscopic and HPLC grade solvents (Burdick and Jackson) were used for the solvatochromic studies. Film thicknesses were measured using an alpha step instrument. Raman spectra were obtained using excitation at 785 nm laser and a Raman microscope (Kaiser Optical Systems). Fabrication of a polymer-layer protected PDA film A typical procedure for the preparation of a protected sensor film is as follows. A thin polymer film ( ca. 1.0 μm) was prepared on a glass substrate by spin-coating a viscous polymer solution containing 10,12-pentacosadiynoic acid (PCDA, 40 mg ml −1 ) and PS (Mw: 280,000 g mol −1 , 5 wt%). The polymer film was then irradiated with a hand-held UV lamp (254 nm, 1 mW cm −2 , 3 min) to induce photopolymerization of PCDA molecules. A readily available photomask, printed on a transparent polymer film, was used to generate PDAs only in the UV-exposed areas. On to the photoirradiated PS film was spin-coated a methanol solution of PAA (Mw: 450,000 g mol −1 , 8 wt%). The thickness of the PAA-protected film was found to be ca. 2.5 μm. Solubility test of a polymer film in an organic solvent A thin polymer film used as a protective layer was prepared on a glass substrate (2.5 × 2.5 cm 2 ) by spin-coating a polymer (PAA, PVC, PVP, PMMA and so on) solution. The polymer-coated glass substrate was incubated in the test solvent for 10 min and placed in a fume hood for 5 min. The weight of the glass substrate was determined before and after incubation in the solvent. Three independent measurements were made and the average value was used. Measurement of colorimetric transition power A thin PS film ( ca. 1.0 μm thickness) containing PCDA (40 mg ml −1 ) was prepared and UV irradiated (254 nm, 1 mW cm −2 , 3 min) to generate a blue coloured PDA film. The film was exposed to a test solvent and the red intensity values of 10 different spots on the solvent-treated film were extracted using the Adobe Photoshop program. How to cite this article: Lee, J. et al. A protective layer approach to solvatochromic sensors. Nat. Commun. 4:2461 doi: 10.1038/ncomms3461 (2013).